Rhodium-catalyzed intermolecular enantioselective Alder–ene type reaction of cyclopentenes with silylacetylenes The Alder–ene type reaction between alkenes and alkynes provides an efficient and atom-economic method for the construction of C-C bond, which has been widely employed in the synthesis of natural products and other functional molecules. The intramolecular enantioselective Alder-ene cycloisomerization reactions of 1,n-enynes have been extensively investigated. However, the intermolecular asymmetric version has not been reported, and remains a challenging task. Herein, we describe a rhodium-catalyzed intermolecular enantioselective Alder-ene type reaction of cyclopentenes with silylacetylenes. A variety of chiral (E)-vinylsilane tethered cyclopentenes bearing one quaternary carbon and one tertiary carbon stereocenters are achieved in high yields and enantioselectivities. The reaction undergoes carbonyl-directed migratory insertion, β-H elimination and desymmetrization of prochiral cyclopentenes processes. The production of synthetically valuable products from readily accessible substrates in a redox-neutral, atom- and step-economical approach is a long-standing goal in organic synthesis. The Alder-ene type reaction comprises a particularly efficient subset of this target [1] , [2] , [3] , [4] , [5] , [6] , which provides an appealing tool to construct C–C bond. Over the past decades, transition metal-catalyzed intramolecular enantioselective Alder-ene type cycloisomerization reactions of 1,6-enynes or 1,7-enynes have been extensively investigated for the rapid assembly of chiral five- or six membered carbo- and hetero-cyclic frameworks (Fig. 1a ) [7] , [8] , [9] , [10] , [11] , [12] , [13] , [14] , [15] , [16] , [17] . However, the intermolecular Alder-ene reactions were mainly confined to less-hindered terminal alkenes [18] , [19] , [20] , [21] , [22] , [23] , [24] , [25] , and the studies on internal alkenes have rarely been reported [26] , [27] . Very recently, Trost and coworkers successfully implemented ruthenium-catalyzed intermolecular alkene–alkyne coupling reactions with well-designed vinyl boronate compounds to synthesize boron-functionalized 1,4-dienes (Fig. 1b ) [28] , [29] , in which the boron substituent played a vital role to facilitate the transformations. However, the intermolecular enantioselective Alder-ene type reaction remains an unexplored territory. Fig. 1: Transition metal-catalyzed Alder-ene type reaction. a Intramolecular enantioselective Alder-ene type cycloisomerization reaction (well-developed). b Intermolecular Alder-ene type reaction of internal alkenes (Trost’s work). c Intermolecular enantioselective Alder-ene type reaction (this work). Full size image All-carbon chiral quaternary stereocenters are fundamental structural motifs present in natural products and pharmaceuticals, which could improve the metabolic stability and target selectivity of biologically active compounds [30] . However, the synthesis of chiral quaternary carbon centers is a challenging task, especially those that are not formed at the direct reaction site [31] , [32] , [33] , [34] , [35] , [36] , [37] , [38] , [39] , [40] , [41] . Asymmetric desymmetrization of prochiral compounds or meso-compounds offers a commendable synthetic tool for achieving this objective [42] , [43] , [44] , [45] , [46] , [47] , [48] , [49] , [50] , [51] , [52] , [53] , [54] . Herein, we describe an asymmetric desymmetrization of prochiral cyclopentenes with silylacetylenes enabled by rhodium-catalyzed intermolecular enantioselective Alder-ene type reaction. This protocol allows access to chiral (E)-vinylsilane tethered cyclopentenes bearing one quaternary carbon and one tertiary carbon stereocenters in high yields and enantioselectivities (Fig. 1c ). Reaction optimization We commenced our studies with the employment of N,1-diphenylcyclopent-3-ene-1-carboxamide 1a and triisopropylsilylyne 2a as the model substrates. 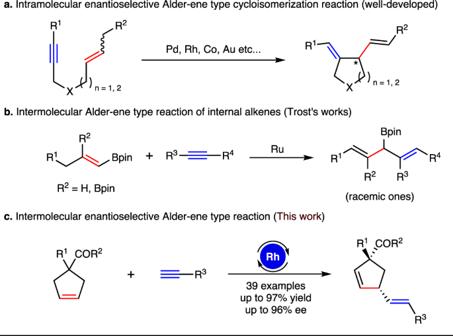Fig. 1: Transition metal-catalyzed Alder-ene type reaction. aIntramolecular enantioselective Alder-ene type cycloisomerization reaction (well-developed).bIntermolecular Alder-ene type reaction of internal alkenes (Trost’s work).cIntermolecular enantioselective Alder-ene type reaction (this work). After considerable screening of the reaction parameters (see the Supplementary Table 1 for details), the desired product 3a was obtained in 96% yield and 95% ee with [Rh(COD)OMe] 2 as the catalyst, phosphoramidite L6 as the ligand, PhMe 2 CCO 2 H and NaBARF as the additives in DCM at 80 °C (Table 1 , entry 1). The P,P-ligands L1 , L2 and N,P-ligand L3 inhibited the transformation (entry 2). Phosphoramidite ligands L4 and L5 performed this reaction in less efficiency (entries 3 and 4). Rh(COD) 2 OTf and [Rh(COD)Cl] 2 gave inferior results compared with [Rh(COD)OMe] 2 , [Cp*RhCl 2 ] 2 and Pd(dba) 2 delivered trace amount yield of product 3a (entries 5–8). AcOH and PhCO 2 H offered 3a in diminished enantioselectivities (entries 9 and 10), and no product was detected in the presence of TsOH (entry 11). Using other additives, such as AgSbF 6 and AgPF 6 could not perform this transformation as well as NaBARF (entries 12 and 13). Conducting the reaction in CHCl 3 and toluene led to lower yields and enantioselectivities (entries 14 and 15), and the reaction was completely suppressed in THF (entry 16). Table 1 Effect of reaction parameters a . Full size table Substrate scope With the optimized reaction conditions in hand, we then explored the generality of this rhodium-catalyzed intermolecular enantioselective Alder-ene type reaction (Fig. 2 ). Various aryl and heteroaryl substituted cyclopentenes (see the Supplementary Methods for details) performed the reactions well, affording the products 3b-3k in 90–94% ee. Replacing the aryl groups with a benzyl group or an alkyl group delivered the products 3l and 3m in 96 and 95% ee. Notably, the substrate 1n containing two alkene moieties, performed the reaction selectively with the endocyclic double bond to give the product 3n in 84% yield with 92% ee. The amino substituted cyclopentene 1o was also suitable substrate for this transfomation, furnishing chiral α-amino acid derivative 3o in 93% ee. N-benzylcyclopent-3-ene-1-carboxamide (R 1 = H) offered the desired product 3p in 90% yield and 94% ee. Fig. 2: Substrate scope. Reaction conditions: 1a (0.10 mmol), 2a (0.30 mmol), [Rh(COD)OMe] 2 (2.5 mol%), L6 (6.0 mol%), PhMe 2 CCO 2 H (60 mol%), NaBARF (10 mol%), DCM (1.0 mL), 80 o C, 36 h, under argon. Isolated yields, d.r. > 20:1, E/Z > 20:1, determined by 1 H NMR analysis. The ee values were determined by chiral HPLC analysis. a [Rh(COD)OMe] 2 (5.0 mol%) , 72 h. b 72 h. c [Rh(COD)OMe] 2 (5.0 mol%). d [Rh(COD)Cl] 2 (5.0 mol%), L5 (12 mol%), Ph 3 CCO 2 H (60 mol%), NaBARF (20 mol%), d.r. > 20:1, Z/E > 20:1. Full size image Subsequently, the compatibilities of amide moiety were investigated, and the products 3q-3w with aryl and alkyl groups were achieved in 86–94% ee. The substrate 1x with tertiary amide group gave 3x in 63% yield with 96% ee under slightly modified conditions. Besides, the enantioenriched spirolactam 3y could also be synthesized in 78% yield and 90% ee. Ester or ketone groups substituted cyclopentenes proceeded this reaction efficiently, affording the products 3z-3ad in 72–93% yields with 90–93% ee. When substrate 1ae was subjected to the standard reaction conditions, no desired product 3ae was detected. After checking the character of cyclopentenes, we then turned our attention to the scope of alkynes. 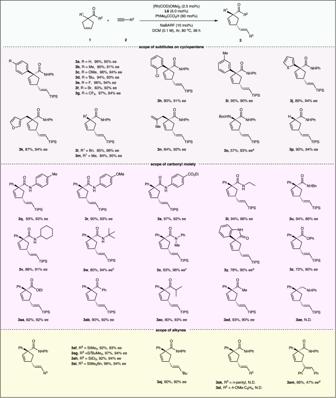Fig. 2: Substrate scope. Reaction conditions:1a(0.10 mmol),2a(0.30 mmol), [Rh(COD)OMe]2(2.5 mol%),L6(6.0 mol%), PhMe2CCO2H (60 mol%), NaBARF (10 mol%), DCM (1.0 mL), 80oC, 36 h, under argon. Isolated yields, d.r. > 20:1, E/Z > 20:1, determined by1H NMR analysis. The ee values were determined by chiral HPLC analysis.a[Rh(COD)OMe]2(5.0 mol%),72 h.b72 h.c[Rh(COD)OMe]2(5.0 mol%).d[Rh(COD)Cl]2(5.0 mol%),L5(12 mol%), Ph3CCO2H (60 mol%), NaBARF (20 mol%), d.r. > 20:1, Z/E > 20:1. 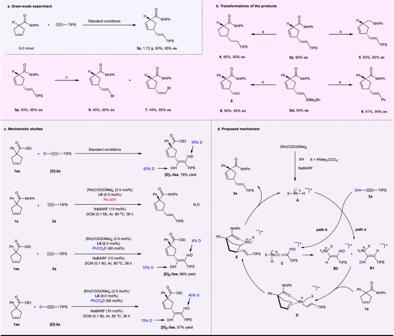Fig. 3: Further studies on the reaction. aGram-scale experiment.bTransformations of the products.aPd/C (10 wt %), B2(OH)4, H2O, DCM, rt.bLiAlH4, 1,4-dioxane, 0oC-80oC, 15 h.cNBS, Ag2CO3, HFIP, rt, 2 h.dTFA, DCM, 60oC, 12 h.ePd(dba)2, TBAF·3H2O, Iodobenzene, THF, rt, 24 h.cMechanistic studies.dProposed mechanism. The reactions proceeded smoothly with diverse silylacetylenes, delivering products 3af-3ai in 93–94% ee. In addition, sterically hindered alkyl alkyne was also proved to be qualified for this reaction, as demonstrated by the formation of product 3aj with 90% ee. Unfortunately, simple alkyl and aryl substituted acetylenes were not yet compatible with the reaction system to give the desired products 3ak and 3al . The 1-heptyne caused the reaction to become confusing, 4-ethynylanisole offered a branched byproduct in a very low yield (see Supplementary Note 1 for details). The internal alkyne biphenylacetylene could participate in this transformation to afford product 3am in 66% yield with 47% ee. The absolute configuration of the product was confirmed by the X-ray analysis of the compound from iododesilylation of 3f (see Supplementary Note 2 for details). Gram-scale experiment and further transformations of the products To demonstrate the synthetic utility of this reaction, a gram-scale experiment (Fig. 3a ) and further transformations of the products 3p and 3ai were carried out (Fig. 3b ). Product 3p (1.72 g) could be synthesized in 93% yield and 95% ee on a 5.0 mmol scale under the standard conditions. A palladium-catalyzed hydrogenation reaction converted 3p to compound 4 in 95% yield. The selective reduction of the amide group of 3p using LiAlH 4 afforded compound 5 in 93% yield. Moreover, compound 3p could be decorated with NBS to give bromination compounds 6 in 40% yield and 7 in 45% yield, respectively. The desilylation of 3ai with TFA offered compound 8 in 94% yield. Arylated product 9 could be constructed through palladium-catalyzed Hiyama cross-coupling reaction, maintaining the E/Z-stereochemistry and enantioselectivity. Fig. 3: Further studies on the reaction. a Gram-scale experiment. b Transformations of the products. a Pd/C (10 wt %), B 2 (OH) 4 , H 2 O, DCM, rt. b LiAlH 4 , 1,4-dioxane, 0 o C-80 o C, 15 h. c NBS, Ag 2 CO 3 , HFIP, rt, 2 h. d TFA, DCM, 60 o C, 12 h. e Pd(dba) 2 , TBAF·3H 2 O, Iodobenzene, THF, rt, 24 h. c Mechanistic studies. d Proposed mechanism. Full size image Mechanistic investigations To gain insight into the mechanism of this reaction, several control experiments and deuterium-labeling experiments were carried out (Fig. 3c ). When [D]-2a was employed, the reaction resulted in [D] 1 -3aa with 63% D atom at β-position to the TIPS group and 35% D atom at α-position. This result implied that a metal vinylidene intermediate could be involved [55] , [56] , [57] . The reaction was drastically prohibited in the absence of the acid. Conducting the reaction with PhCO 2 D provided [D] 2 -3aa with 10% D atom at β-position to the TIPS group and 6% D atom at α-position, which indicated that the acid may work with the rhodium(I) to catalyze this reaction by the formation of RhH species. The generation of product [D] 3 -3aa from [D]-2a with PhCO 2 D further supported the hypothesis. Based on the above experiment results and previous works [45] , [46] , [47] , [55] , [56] , [57] , [58] , [59] , [60] , a possible reaction pathway is depicted in Fig. 3d with 1a and 2a as the model substrates. Oxidative addition of rhodium(I) into PhMe 2 CCO 2 H generates RhH species A , and the presence of NaBARF plays a pivotal role for the generation and stabilization of this cationic rhodium complex [59] , [60] . Regioselective alkyne insertion into the species A forms vinylrhodium intermediate B1 directly (path a). On the other hand, η 2 -coordination of the alkyne to the species A followed by rearrangement generates an η 1 -vinylidenerhodium species C [55] , [56] , [57] , which could produce intermediate B2 via migratory insertion (path b). Coordination of B1 or B2 to the double bond of 1a directed by carbonyl group forms the rhodium(III) intermediate D [45] , [46] , [47] , [58] , which undergoes syn-migratory insertion to afford the intermediate E . Subsequent β-hydride elimination of E offers the desired product 3a . In conclusion, we have described a rhodium-catalyzed intermolecular enantioselective Alder-ene/desymmetrization reaction of prochiral cyclopentenes with alkynes directed by carbonyl group. This method provides a practical route for the synthesis of chiral (E)-vinylsilane tethered cyclopentenes bearing one quaternary carbon and one tertiary carbon stereocenters in high efficiency and atom-economy. Further studies on the reaction mechanism and expansion of the asymmetric intermolecular Alder-ene type reactions are underway in our laboratory. General procedure for the rhodium-catalyzed intermolecular enantioselective Alder-ene type reaction of cyclopentenes with silylacetylenes To an oven-dried 10-mL Schlenk tube equipped with a teflon-coated magnetic stir bar was added 1a (26.3 mg, 0.100 mmol, 1.00 equiv), [Rh(COD)OMe] 2 (1.2 mg, 2.5 mol%), L6 (2.7 mg, 6.0 mol%), NaBARF (8.9 mg, 10 mol%) and PhMe 2 CCO 2 H (10 mg, 60 mol%). The vial was thoroughly flushed with argon, and 2a (54.7 mg, 0.600 mmol, 3.00 equiv), as well as DCM (1.0 mL) was added under argon atmosphere. Then the reaction mixture was stirred at 80 °C for 36 h. After the reaction vessel was cooled to room temperature, the solution was concentrated in vacuum and purified by careful chromatography on silica gel (PE/EA = 50/1) to afford the desired product 3a .